Towards graphyne molecular electronics α-Graphyne, a carbon-expanded version of graphene (‘ carbo -graphene’) that was recently evidenced as an alternative zero-gap semiconductor, remains a theoretical material. Nevertheless, using specific synthesis methods, molecular units of α-graphyne (‘ carbo -benzene’ macrocycles) can be inserted between two anilinyl (4-NH 2 -C 6 H 4 )-anchoring groups that allow these fragments to form molecular junctions between gold electrodes. Here, electrical measurements by the scanning tunnelling microscopy (STM) break junction technique and electron transport calculations are carried out on such a carbo -benzene, providing unprecedented single molecule conductance values: 106 nS through a 1.94-nm N–N distance, essentially 10 times the conductance of a shorter nanographenic hexabenzocoronene analogue. Deleting a C 4 edge of the rigid C 18 carbo -benzene circuit results in a flexible ‘ carbo -butadiene’ molecule that has a conductance 40 times lower. Furthermore, carbo -benzene junctions exhibit field-effect transistor behaviour when an electrochemical gate potential is applied, opening the way for device applications. All the results are interpreted on the basis of theoretical calculations. The revolution in carbon materials can be illustrated by a series of breakthroughs, from the discovery of zero-dimensional carbon fullerenes (C 60 , 1982) [1] to that of one-dimensional (1D) carbon nanotubes (CNTs, 1991) [2] , and most recently of two-dimensional (2D) graphene sheets [3] . The interest they have attracted is largely due to their unique electrical properties. The extremely high conductivity of graphene is theoretically rationalized as a consequence of its band structure exhibiting a so-called Dirac cone, supposed to be one of the unique features of graphene allowing long-range ballistic transport [4] . Recently, however, first-principles calculations have shown that α-graphyne, a theoretical carbon allotrope composed of ‘giant’ hexagonal units made of graphenic sp 2 and nongraphenic sp carbon atoms in a 1/3 ratio ( Fig. 1 ), also exhibits Dirac cones [5] , [6] , implying that structures containing α-graphyne units could be key to the advent of another generation of carbon electrical materials [2] , [7] . α-Graphyne [8] , whose appealing structure was first proposed by Baughman in 1987 for possible electronic, optical and mechanical properties [2] , [4] , is actually the total carbo -mer of graphene (‘ carbo -graphene’): it indeed arises from the insertion of C 2 units into each bond of graphene by formal carbo -merization. This process, defined in 1995 at the molecular level [9] , was also more recently theoretically applied to carbon allotropes of lower dimensionality such as CNTs [10] , [11] , [12] , or fullerenes [13] . Although such carbo -allotropes remain unknown, α-graphyne can be viewed as an assembly of fused carbo -benzene rings [14] . The highly symmetrical ‘carbon- and π-electron-enriched’ structure of these C 18 macrocycles has naturally prompted much effort for their experimental synthesis [15] , and theoretical analysis of their fundamental electronic properties, in particular electron delocalization and aromaticity [16] . 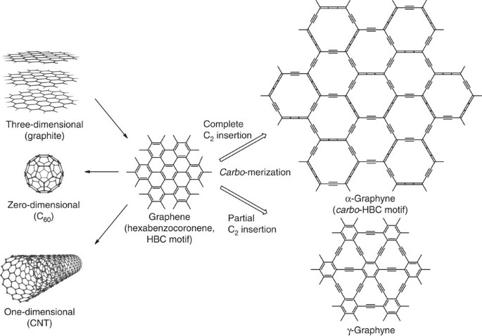Figure 1: Examples of carbon allotrope materials. Fullerenes (C60) are zero-dimensional carbon quantum dots; CNTs are 1D carbon tubules obtained when a 2D carbon sheet of graphene is rolled up; graphynes are ‘expanded’ forms of graphene, where C2units are inserted intosp2C–sp2C bonds of the parent C6rings, either partially, in γ-graphyne, or totally, in α-graphyne (carbo-graphene). Figure 1: Examples of carbon allotrope materials. Fullerenes (C 60 ) are zero-dimensional carbon quantum dots; CNTs are 1D carbon tubules obtained when a 2D carbon sheet of graphene is rolled up; graphynes are ‘expanded’ forms of graphene, where C 2 units are inserted into sp 2 C– sp 2 C bonds of the parent C 6 rings, either partially, in γ-graphyne, or totally, in α-graphyne ( carbo -graphene). Full size image Similarly to chemical analogy (that is, atom or group replacement, for example, replacing carbon with silicon), carbo -merization (by C 2k expansion) is a systematic means for creating molecular diversity, and therefore a natural tool for investigating structure–activity relationships. An emerging research gap in graphene science—going beyond graphene technology—is the need for structural generalization. This has been recently addressed at the experimental level by considering chemical analogues, for example, silicene [17] and related composite inorganic 2D materials [18] , as well as partial carbo -mers, for example, γ -graphyne. Total carbo -mers of graphene such as α-graphyne or α-graphdiyne have been considered at the theoretical level only. Nevertheless, a variation of the graphene structure is currently more realistically addressed by restricting the infinite sheet to fragments of controlled size and shape: nanoribbons, flakes, functional nanographenes [19] , small polycyclic aromatic hydrocarbons, oligophenylene and ultimately the benzene molecule itself [20] . In their seminal paper ‘Electron Transport in Single Molecules: From Benzene to Graphene’, Chen and Tao [20] justify the relevance of the continuity between the single molecule and the corresponding infinite material made of fused molecular units. The same principle may apply to carbo -benzenes, thus making the study of known single carbo -benzenic molecules relevant to gaining insight into the still to be realized carbo -graphene material. In this contribution, the charge transport properties, and in particular the single molecule conductance (SMC) of carbo -meric molecules (considered as the ‘basic units’ of infinite α-graphyne), are explored both experimentally by scanning tunneling microscopy (STM) break junction techniques, and theoretically by NEGF-DFT (nonequilibrium Green’s function-density functional theory) calculations. Two carbo -meric molecules, differing by the nature of their conjugated bridge (macrocyclic in one case and acyclic in the other), are considered. In a step towards device applications, the electrochemical gating effect on the molecular junction conductance is also investigated. Conductance of the carbo -benzene A To measure molecular junction conductance, molecules have to be functionalized by anchoring groups to be wired into the metal junctions. It has been reported that the amine (NH 2 ) functionality is a highly efficient anchoring group for SMC studies, as it can form molecular junctions with small fluctuations in conductance (because of its specific coupling with gold electrodes), and thus reduce the variability in binding geometries [21] . Therefore, previously described diamino-functionalized carbo -meric molecules were selected for the present study [22] , namely the ideally centrosymmetric (quadrupolar) para -dianilinyl- carbo -benzene A ( Fig. 2a ), and the di-anilinyl-dibutatrienylacetylene (DBA) B ( Fig. 2b ), in which the α-graphynic macroaromatic C 18 circuit of A (which can also be regarded as a hexagonal carbocyclic alternative to the C 16 N 2 heterocycle of square-shaped porphyrins) [23] is replaced by a linear (acyclic) π-conjugated C 10 chain, namely the carbo -mer of the n -butadiene core. 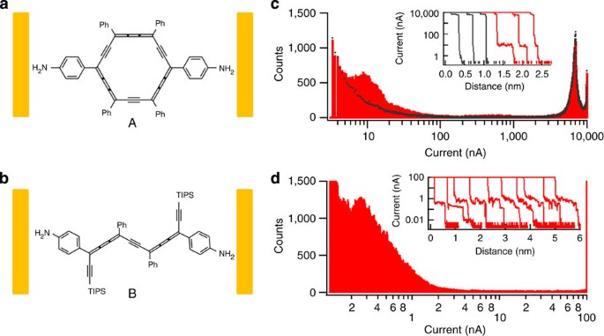Figure 2: Single molecule conductance measurements forcarbo-benzene andcarbo-n-butadiene. (a,b) Structures ofcarbo-benzeneAandcarbo-n-butadiene (DBA)B, respectively, trapped in STM metal junctions. TIPS group=TriIsoPropylSilyl=Si(iPr)3. (c) All-data histogram constructed from 3,000 current–distance traces for thecarbo-benzeneA(red) and control experiments without adding target molecules (black) measured at a bias voltage of 0.1 V. Inset shows sample individual traces for thecarbo-benzeneA(red) and control experiments (black). (d) All-data histogram constructed from 3,000 current–distance traces for thecarbo-n-butadieneBmeasured at a bias voltage of 0.1 V. Inset shows sample individual traces for DBA. Figure 2: Single molecule conductance measurements for carbo -benzene and carbo-n -butadiene. ( a , b ) Structures of carbo -benzene A and carbo-n -butadiene (DBA) B , respectively, trapped in STM metal junctions. TIPS group=TriIsoPropylSilyl=Si(iPr) 3 . ( c ) All-data histogram constructed from 3,000 current–distance traces for the carbo -benzene A (red) and control experiments without adding target molecules (black) measured at a bias voltage of 0.1 V. Inset shows sample individual traces for the carbo -benzene A (red) and control experiments (black). ( d ) All-data histogram constructed from 3,000 current–distance traces for the carbo-n -butadiene B measured at a bias voltage of 0.1 V. Inset shows sample individual traces for DBA. Full size image Measurements of charge transport through single carbo -meric molecular junctions were experimentally realized using the STM break junction technique, where an STM tip and a metal substrate function as two electrodes connecting to the two anchoring groups of the molecule [24] , [25] , [26] . In STM break junction experiments, approaching and separating the tip and substrate electrodes allow the formation of an atomically thin metal junction [26] , [27] . Electron transport through such an atomic wire can approach the ballistic transport limit manifested by the observation of a quantized conductance of value 1 G 0 , ( G 0 =2 e 2 / h =77,500 nS, where e and h are the electron charge and Planck’s constant, respectively) [28] , which is revealed as steps in current–distance traces ( Fig. 2c , inset, black) and a peak in the current histogram near 8,000 nA ( Fig. 2c , black). After the metal junction breaks, exponentially decaying traces are expected unless there are molecules trapped in the gap between the two electrodes. If conducting molecules are connected between the two electrodes by their anchoring groups, a molecular junction forms and current steps, which are usually orders of magnitude smaller than the G 0 value, are observed. These small current steps (≈10 nA) correspond to molecular junction conductance [26] . Some current–distance traces for the carbo -benzene A -mediated junction ( Fig. 2c inset, red) clearly show characteristic current steps around 10 nA at a bias voltage of 0.1 V. In addition to quantum conductance current peak ( G 0 , ≈7,500 nA) associated with Au atomic junctions [26] , the histogram, generated using all traces without data selection, also shows a current maximum at 10 nA, corresponding to a SMC of ca 100 nS. The experimentally determined SMC value for the carbo -benzene A is 106±10 nS, averaged from different experiments measured on different days. Similar results were obtained from two samples of A prepared by two different syntheses. This value represents the largest reported SMC of any amine-anchored molecule of similar length, such as a porphyrin or a highly conjugated oligophenylene-ethynylene ( Supplementary Table 1 ). In particular, the SMC of the α-graphyne molecular fragment A studied here is much larger (106 nS through 1.94 nm) than that of the shorter, and therefore in principle more conductive, graphene molecular fragment hexabenzocoronene (HBC) measured with the same technique (14 nS through 1.4 nm) [29] . The conductance of carbo -benzene can also be compared with another class of molecules previously studied by our group [27] . The conductance of the dyes pararosaniline and malachite green depends on the pH of the solution they are found in. The highest conductance of the dyes was measured for pararosaniline at pH=5.5 to be 71.6 nS. Not only is the conductance higher for carbo -benzene, but carbo -benzene has a N–N distance that is more than twice the N–N distance in pararosaniline (19.4 versus 9.6 Å, respectively). To shed light on the superior conducting properties of the carbo -benzene A , the electron transport was modelled with the NEGF technique in combination with DFT [30] , [31] . The NEGF-DFT approach was previously employed to interpret STM experiments, and the details of the technique can be found in refs 27 , 32 , 33 and in the Methods section. To briefly summarize the method, a model was devised for a two-probe system consisting of a molecule bridging a gap between two semi-infinite metallic electrodes. This two-probe system is partitioned into the periodic left and right electrodes, and the nonperiodic molecular region (see Fig. 7 ). The NEGF-DFT formalism relies on a self-consistent electronic structure calculation from which can be extracted the transmission function—the probability that an electron with a given energy will pass from the left electrode, through the molecule and into the right electrode. Using a Landauer–Büttiker approach [32] , [34] , [35] , the transmission function can then be integrated for an appropriate energy window to obtain the current that would pass through the molecule at that particular bias. The path of the electron is here assumed to occur exclusively through the NH 2 ends (although formally possible in principle [36] , conduction through the weakly binding, weakly competing carbon centres is not considered). Figure 7: Two-probe structure used for the NEGF-DFT electron transport calculations. The effects of the electrodes on the central region are included in the self-energies, ∑ 1,2 . 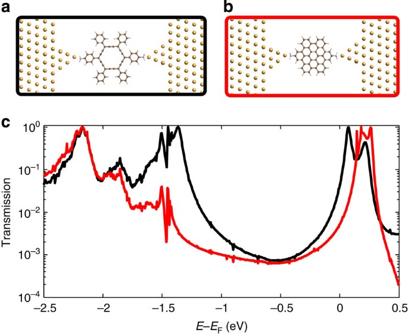Figure 3: Structures and transmission spectra ofcarbo-benzene and graphene flake molecular junctions. (a,b) Two-probe structures forcarbo-benzeneAand a HBC graphene flake, respectively. (c) The transmission spectra corresponding to these systems: black forcarbo-benzene, red for graphene flake. Thecarbo-benzene has a considerably smaller HOMO–LUMO gap, resulting in higher transmission over a wide energy range. Full size image Figure 3 shows the computed transmission spectra for electron transport through the carbo -benzene A (black) and through a HBC graphene flake (red) similar to the one measured in ref. 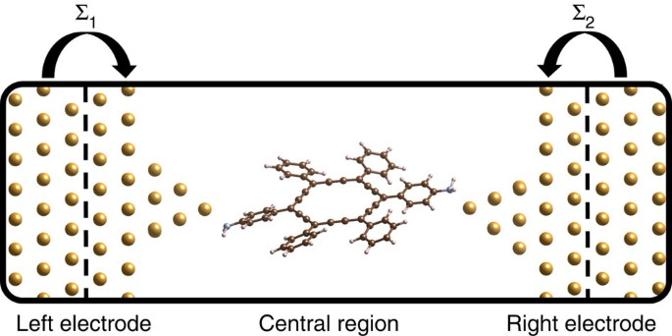Figure 7: Two-probe structure used for the NEGF-DFT electron transport calculations. The effects of the electrodes on the central region are included in the self-energies, ∑1,2. 25 . The tall transmission peaks near −1.5 and 0.1 eV represent resonant transport through the highest occupied molecular orbital (HOMO) and the lowest unoccupied molecular orbital (LUMO) levels of the carbo -benzene, respectively. The actual Fermi level of the electrodes in the experiment is somewhere in between these levels, where resonant tunnelling can occur through the tails of the transmission peaks. The graphene flake has a larger HOMO–LUMO gap and one can see that the transmission through the carbo -benzene core is higher than through the graphene flake. This means that, at energies between the resonant transmission peaks, the transmission does not decay as rapidly with distance in the carbo -benzene as it does in the graphene flake. Carbo -benzene is a more efficient molecular conductor even though it is ~40% longer than the graphene flake. Figure 3: Structures and transmission spectra of carbo -benzene and graphene flake molecular junctions. ( a , b ) Two-probe structures for carbo -benzene A and a HBC graphene flake, respectively. ( c ) The transmission spectra corresponding to these systems: black for carbo -benzene, red for graphene flake. The carbo -benzene has a considerably smaller HOMO–LUMO gap, resulting in higher transmission over a wide energy range. Full size image Conductance of the carbo-n -butadiene B The SMC of the carbo -benzene A was then compared with that of the carbo -butadiene (DBA) B . Topologically, these two molecules present the same type of π-conjugated chains between the two NH 2 end groups, either in twin pathways inside the macroaromatic circuit of A , or as a single DBA chain in the acyclic wire of B . The STM break junction experiments were carried out under the same conditions, and sample individual current–distance traces and corresponding all-data histograms, constructed from 3,000 traces without selection, are illustrated in Fig. 2d . The SMC of DBA B was determined to be 2.7 nS from the current maximum of 0.27 nA in the histogram ( Fig. 2d ) for a bias voltage of 0.1 V, by averaging more than 10 histograms from different experiments performed on different days, and the overall value (2.7±0.4 nS) appears to be ~40 times smaller than the conductance of the carbo -benzene A , in spite of their strong similarity in size and local structure (the two molecules have the same NH 2 -anchoring groups and the same type of conjugated chains between them). Beyond the duplication of the π-conduction pathways in A versus B , a key difference is that the carbo -benzene A has a planar and rigid macroaromatic core, while the carbo -butadiene B presents a flexible n –π-conjugated DBA skeleton (experiments were carried out at 294 K). When passing from A to B , cutting off the 18 π-electron cyclic conjugation makes the molecule lose its rigid planar conformation: the DBA core can indeed adopt numerous geometries including nonvanishing torsional angles so that the overlap of the π-orbitals from one side of the molecule to the other decreases significantly. This is consistent with previous reports showing that the SMC decreases with increasing twist angle in a series of biphenyl molecules [21] , [37] . The current peak in the histogram ( Fig. 2d ) is very broad, stretching from the central peak of 0.27 nA, up to over 1 nA, thus indicating that there is a wide range of junction conductances, which could be because of the conformational variation of the flexible skeleton of the DBA B in junctions. 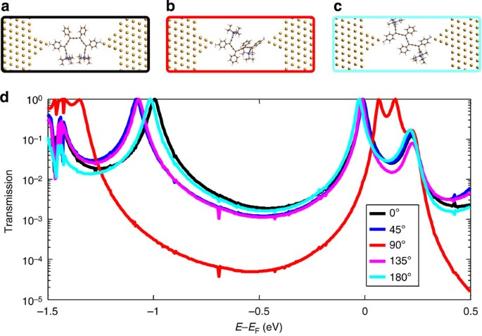NEGF-DFT transport calculations were performed on different conformations of the DBA molecule having different dihedral rotational angle values about the central C–C≡C–C edges of the core. Figure 4: Structures and transmission of DBA having various dihedral angles. (a–c) Two-probe structures for DBA having dihedral (twist) angles around central C–C≡C–C segment of 0°, 90° and 180°, respectively. (d) Transmission spectra for DBA for various dihedral angles. Figure 4 shows the transmission spectra for DBA conformations with various dihedral (twist) angles. The significant difference is that the HOMO–LUMO gap increases as the molecule loses planarity, and this results in lower transmission values between them, which is dramatically apparent when the transmission is plotted on a logarithmic scale. Even a dihedral angle of 45° (or 135°) results in a noticeably lower transmission at certain energies, and a rotation of 90° can lead to a reduction of transmission by two orders of magnitude (although it is unlikely that the molecule would adopt conformations with dihedral angles so far from being planar—see Fig. 8 for potential energy profile). It is noteworthy that this decrease in transmission is obtained by rotation about a single bond of the DBA core, among all the freely rotating bonds of the molecule. At 294 K, slight deviations from planarity in several bonds can result in a drastic overall reduction in transmission, which explains the observed 40-fold reduction in SMC of B compared with A . In short, the stiffness of the aromatic C 18 macrocycle of A , which maintains its planarity, is responsible for the superior conductance compared with less rigid molecules of similar length (like B ). Figure 4: Structures and transmission of DBA having various dihedral angles. ( a – c ) Two-probe structures for DBA having dihedral (twist) angles around central C–C≡C–C segment of 0°, 90° and 180°, respectively. ( d ) Transmission spectra for DBA for various dihedral angles. Full size image Figure 8: Structure of DBA and rotational energy profile. ( a ) Isolated DBA molecule used for dihedral angle potential energy calculations. 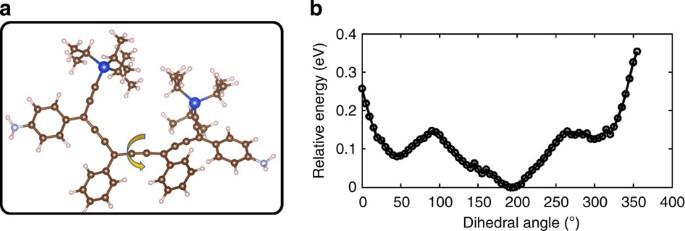Figure 8: Structure of DBA and rotational energy profile. (a) Isolated DBA molecule used for dihedral angle potential energy calculations. The yellow arrow shows the C–C≡C–C segment that the molecule was rotated around. (b) Relative energy as a function of dihedral angle. The yellow arrow shows the C–C≡C–C segment that the molecule was rotated around. ( b ) Relative energy as a function of dihedral angle. Full size image Gating for the carbo -benzene A The ability to control charge transport via an external perturbation is prerequisite for the design of useful molecular electronic devices [38] . This can be achieved by using an external potential, called electrochemical gating [38] , [39] , [40] , that shifts the frontier molecular orbitals (HOMO/LUMO) with respect to the Fermi level of the Au tip and substrate [39] , [41] . The resulting change in the energy separation (alignment) between the HOMO/LUMO and the Fermi level of the electrodes yields a field-effect transistor function [29] . The electrochemical gating measurements are illustrated in Fig. 5 . In an STM break junction configuration, a carbo -benzene molecule A was wired between the tip and substrate electrodes, acting as the ‘source’ and the ‘drain’ electrodes, respectively. The reference electrode, that is, the ‘gating electrode’, was used to tune the working electrode potentials and molecular orbital energies. When the frontier molecular orbitals of the molecule in the junction are modulated to approach the Fermi level of the source and drain electrodes, an increase in the charge transport through the molecular junction is a priori expected. The gating effect was thus investigated by measuring the SMC of carbo -benzene junctions at different gating potentials, while keeping the bias voltage (the potential difference between the source and drain) constant. An ionic liquid of wide potential window (trihexyltetradecyl-phosphonium-bis(2,4,4-trimethylphenyl)phosphinate) was used as the electrochemical gating electrolyte. A few sample current–distance traces, measured at a sample (drain) potential of −0.1, −0.6 and −1.3 V and a bias voltage of 0.1 V are shown in Fig. 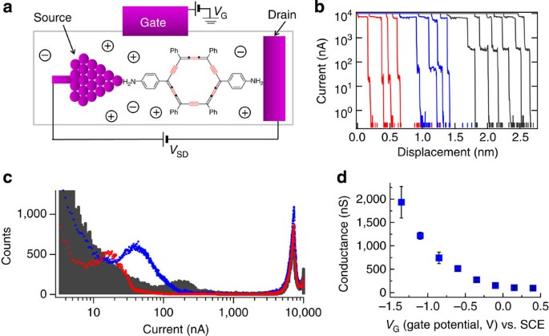5 , along with all-data point current histograms, constructed from individual traces, without selection. The conductance is also plotted as a function of the gate (sample) potential, clearly showing a gating effect, that is, the increase in the SMC value as the gating potential becomes more negative, with an observed on/off ratio of an order of magnitude (≈15). Figure 5: Single molecule electrochemical gating ofcarbo-benzene in an ionic liquid. (a) Schematics of the gating experiment in an electrochemical STM break junction configuration. (b) Sample individual current–distance traces measured at three gate potentialsEsample=−0.1 V (red), −0.6 V (blue), −1.35 V (dark grey) and a bias voltage of 0.1 V. (c) Current histograms measured atEsample=−0.1 V (red), −0.6 V (blue) and −1.35 V (dark grey), respectively. Bias voltage: 0.1 V. (d) Gated SMC of thecarbo-benzeneAas a function of the gating (sample) potentialVG. Error bars were obtained by averaging 3-10 measurements for each potential. Electrode potential is referred to the saturated calomel electrode (SCE). Figure 5: Single molecule electrochemical gating of carbo -benzene in an ionic liquid. ( a ) Schematics of the gating experiment in an electrochemical STM break junction configuration. ( b ) Sample individual current–distance traces measured at three gate potentials E sample =−0.1 V (red), −0.6 V (blue), −1.35 V (dark grey) and a bias voltage of 0.1 V. ( c ) Current histograms measured at E sample =−0.1 V (red), −0.6 V (blue) and −1.35 V (dark grey), respectively. Bias voltage: 0.1 V. ( d ) Gated SMC of the carbo -benzene A as a function of the gating (sample) potential V G . Error bars were obtained by averaging 3-10 measurements for each potential. Electrode potential is referred to the saturated calomel electrode (SCE). Full size image NEGF-DFT simulations have been carried out to elucidate the gating mechanism. The calculations are similar to those performed to obtain the results displayed in Fig. 3 ; however, a gate effect was simulated by adding a gate-induced electrostatic boundary condition to the system (see Fig. 6a and Methods section). The result of the gate for carbo -benzene is that it shifts the LUMO (and other MOs) with respect to the Fermi level of the electrodes ( Fig. 6b ). 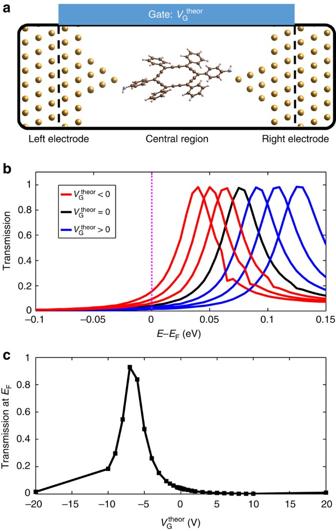Note that the sign convention for a field-effect transistor gate (in calculations) is the opposite of that adopted in an electrochemical gate (in experiment) [39] ; therefore, the sign of V G theor presented here has been reversed so that comparison with experiment can be made more easily. We can see that the application of a negative gate voltage lowers the LUMO energy, bringing it closer to E F , thereby increasing conductance. Figure 6: Gating NEGF-DFT calculation results. (a) Two-probecarbo-benzene structure with a gate electrode added at the boundary of the simulation box (the gate region encompasses the entire central region). (b) Effect of gating on the transmission spectrum nearEF. The LUMO peak is atE−EF=0.075 eV whenVGtheor=0. Positive gate voltages ofVGtheor=1.0, 2.0 and 3.0 V shift the LUMO progressively to the right, while negative voltages ofVGtheor=−1.0, −2.0 and −3.0 V shift the LUMO progressively to the left. (c) Transmission at theEFfor variousVGtheorvalues. Note that the sign of calculatedVGtheorvalues has been reversed to allow for easier comparison with the electrochemical gating measurements inFig. 5ddue to a sign convention difference (see text and ref.39). Figure 6c shows the calculated transmission at E F for different V G theor values. Comparing the range of V G theor =−5 to +5 V, there is good qualitative agreement with Fig. 5d . Note that the magnitude of the V G theor values in Fig. 6c are arbitrary (the results indeed depend on the simulation box size, that is, the distance of the gate from the molecule); however, the theoretical trend does predict that, had it been possible to experimentally apply gate potential values of V G <−1.5 V (in Fig. 5d ), the conductance would go through a maximum as the LUMO would pass through the source-drain bias window, and decrease with more negative V G . Although this was not achieved for carbo -benzene with this experimental set-up, it has been reported for other molecules [42] . Figure 6: Gating NEGF-DFT calculation results. ( a ) Two-probe carbo -benzene structure with a gate electrode added at the boundary of the simulation box (the gate region encompasses the entire central region). ( b ) Effect of gating on the transmission spectrum near E F . The LUMO peak is at E − E F =0.075 eV when V G theor =0. Positive gate voltages of V G theor =1.0, 2.0 and 3.0 V shift the LUMO progressively to the right, while negative voltages of V G theor =−1.0, −2.0 and −3.0 V shift the LUMO progressively to the left. ( c ) Transmission at the E F for various V G theor values. Note that the sign of calculated V G theor values has been reversed to allow for easier comparison with the electrochemical gating measurements in Fig. 5d due to a sign convention difference (see text and ref. 39 ). Full size image Single molecule charge transport properties are probed by STM break junction observations and NEGF-DFT calculations, demonstrating that the macrocyclic conjugation of the carbo -benzene core (the α-graphyne unit) provides superior junction conductance. This effect is a priori compatible with the weak energetic aromaticity of the C 18 carbo -benzene macrocycle ( ca three time less aromatic, and thus less ‘insulating’, than the parent C 6 benzene ring) [16] . The small HOMO–LUMO gap of the carbo -benzene allows the gating of charge transport by shifting the alignment of molecular levels relative to the Fermi energy of the source and drain. Within the electrochemically accessible window, an order of magnitude increase in junction conductance is achieved. These remarkable electrical properties arise from the unique electronic structure of the carbo -benzene macrocycle, provided by the combination of sp and sp 2 carbons, and make molecular fragments of α-graphyne promising for the design of novel classes of carbon materials having potential for device applications. Preparation of the carbo -benzene A and carbo- butadiene B The carbo -meric conductors A and B were prepared according to previously described procedures [22] , the last steps of which are described below (and in Supplementary Fig. 1 ). Preparation of the ‘ p -bis(4-aminophenyl)tetraphenyl- carbo -benzene’ A : 4-[10-(4-aminophenyl)-4,7,13,16-tetraphenylcyclooctadeca-1,2,3,7,8,9,13,14,15-nonaen-5,11,17-triyn-1-yl]aniline: A solution of p -bromo-N,N-bis(trimethylsilyl)aniline (0.38 ml, 1.35 mmol) in tetrahydrofuran (THF) (1 ml) was added slowly at room temperature to a suspension of magnesium turnings (32 mg, 1.32 mmol) in THF (0.5 ml). After the Grignard reagent was formed, the mixture was added to a solution of the key [6]pericyclynedione 1a (see Supplementary Fig. 1 ; prepared in nine steps and 7% yield as described in ref. 2 ) [43] (150 mg, 0.22 mmol) in THF (10 ml) at 0 °C. The stirring was maintained for 2 h at 0 °C, and then overnight at room temperature. After addition of water, the aqueous layer was extracted with diethylether (Et 2 O). The combined organic layers were washed with brine, dried over MgSO 4 and evaporated under reduced pressure. The obtained poorly stable [6]-pericyclynediol 2a was directly used in the reduction step without further purification. The mixture was thus dissolved in dichloromethane (DCM), before addition of SnCl 2 (417 mg, 2.21 mmol), and then in HCl·Et 2 O (2.20 ml, 4.40 mmol) at −78 °C. The reaction mixture was allowed to warm up to room temperature slowly, and the stirring was maintained for 1 h at room temperature, before hydrolytic treatment with aqueous 1 M NaOH (4.6 ml) and stirring overnight. After treatment with brine, the aqueous layer was extracted with DCM. The combined organic layers were dried over MgSO 4 and evaporated under reduced pressure. The residue was purified using silica gel chromatography, eluting first with DCM:THF:acetone in ratios 8:1:1, 7:1.5:1.5, 6:2:2, and then subsequently with THF:acetone. The concentration residue of the collected fractions was washed with pentane to give pure A as a green-gold solid (40 mg, 26% yield for the two steps). 1 H NMR (THF D 8 ): δ =7.23 (d, 3 J HH =8.5 Hz, 4H, m -C 6 H 4 -N), 7.72 (t, 3 J HH =7.5 Hz, 4H, p -C 6 H 5 ), 8.01 (pseudo-t, 3 J HH =7.5 Hz, 8H, m -C 6 H 5 ), 9.23 (d, 3 J HH =8.5 Hz, 4H, o -C 6 H 4 -N), 9.47 (d, 3 J HH =7.5 Hz, 8H, o -C 6 H 5 ). 13 C{ 1 H} NMR (THF D 8 ): δ =101.8 ( C -C 6 H 5 ), 105.8 ( C -C 6 H 4 -N), 115.1 ( m - C 6 H 4 -N), 116.0, 118.2 (C= C = C =C, C– C ≡ C –C), 128.8 ( i - C 6 H 4 -N), 128.8 ( p - C 6 H 5 ), 129.6 ( m - C 6 H 5 ), 130.0 ( o - C 6 H 5 ), 131.8 ( o - C 6 H 4 -N), 140.4 ( i - C 6 H 5 ), 151.0 ( p - C 6 H 4 -N). MS (MALDI-TOF/DCTB): m/z =708.4 [M] + . HRMS (MALDI-TOF/DCTB): m/z calcd for C 54 H 32 N 2 : 708.2565, found: 708.2635. UV–vis (CHCl 3 ): λ max =493 nm ( ε =105,349 l mol −1 cm −1 ) and m.p. (melting point)=180 °C. Preparation of ‘ p -bis(4-aminophenyl)diphenylbis(triisopropylsilyl)- carbo -butadiene B : 4-{12-[4-aminophenyl]-6,9-diphenyl-1,14-bis[tris(propan-2-yl)silyl]tetradeca-3,4,5,9,10,11-hexaen-1,7,13-triyn-3-yl}-aniline: a solution of p -bromo-N,N-bis(trimethylsilyl)-aniline (0.40 ml, 1.42 mmol) in THF (1 ml) was added slowly at room temperature to a suspension of magnesium turnings (33 mg, 1.36 mmol) in THF (0.5 ml). After the Grignard reagent was formed, the mixture was added to a solution of the diketone 1b obtained quantitatively by MnO 2 -mediated oxidation of the corresponding secondary diol (see ref. 1 of the Supplementary Information; 170 mg, 0.23 mmol) in THF (5 ml) at 0 °C. The stirring was maintained for 2 h at 0 °C, and then overnight at room temperature. After addition of water, the aqueous layer was extracted with Et 2 O. The combined organic layers were washed with brine, dried over MgSO 4 and evaporated under reduced pressure. The obtained poorly stable pentaynediol 2b was directly used in the reduction step without further purification. The mixture was thus dissolved in DCM (70 ml), before the addition of SnCl 2 (440 mg, 2.33 mmol), and then in HCl·Et 2 O (2.31 ml, 4.62 mmol) at −78 °C. The temperature was allowed to increase slowly up to −20 °C, affording a red-dark mixture. Aqueous 1 M NaOH (4.8 ml) was then added, and the mixture was allowed to warm up to room temperature while becoming dark blue. After addition of brine, the aqueous layer was extracted with DCM. The combined organic layers were dried over MgSO 4 and evaporated under reduced pressure. The residue was purified using silica gel chromatography (DCM/pentane 1:9, then 2:8) to give B as green-gold solid in 53% yield over two steps. 1 H NMR (THF D 8 ): δ =1.20–1.29 (m, 42H, Si-C H -C H 3 ), 5.30 (bs, 4H, N H 2 ), 6.60–6.65 (m, 4H, m -C 6 H 4 -N), 7.27–7.47 (m, 6H, m -, p -C 6 H 5 ), 7.63–7.68 (m, 4H, o -C 6 H 4 -N), 7.83–7.93 (m, 4H, o -C 6 H 5 ). 13 C{ 1 H} NMR (THF D 8 ): δ =12.4 (Si- C H-CH 3 ), 19.2 (Si-CH- C H 3 ), 99.9, 100.2, 100.3, 100.5, 100.6, 100.8, 101.5, 101.6, 106.1, 106.2, 106.2, 106.6, 106.9 ( C ≡ C –Si and C – C ≡ C–C ), 114.8, 114.9, 115.0 ( m - C 6 H 4 -N), 126.2, 126.2, 126.9, 127.4, 127.5, 127.8, 128.7, 128.7, 129.3, 129.3, 129.4, 129.4, 129.5, 129.8, 129.8, 130.1 ( o -, m -, p - C 6 H 5 and o - C 6 H 4 -N), 137.6, 137.8, 138.5 ( i - C 6 H 5 ), 141.6, 141.8, 141.8 ( i - C 6 H 4 -N), 144.2, 144.3, 144.6 (C= C = C =C), 151.4, 151.6, 151.7 ( p - C 6 H 4 -N). MS (MALDI-TOF/DCTB): m/z : 820.4 [M] + . HRMS (MALDI-TOF/DCTB): m/z calcd for C 56 H 64 N 2 Si 2 : 820.4625, found: 820.4608. UV–vis (CHCl 3 ): λ max =622 nm ( ε =38,654 l mol −1 cm −1 ), 456 (25,009), 379 (20,804) and m.p.(dec)=210 °C. Electrode and sample preparation Before each experiment, Au(111) single crystal disk electrodes (10 mm diameter, 2.0 mm height, from MaTeck, Germany) were first cleaned with piranha solution (H 2 O 2 (30%):H 2 SO 4 (concentrated, 96%)=1:3; (CAUTION: ‘piranha’ solutions are very reactive mixtures! They must be handled with great care; use of protective equipment, such as gloves, goggles and lab coat, is necessary). The electrodes were then rinsed with ultraclean deionized water (Thermoscientific Barnstead Easypure II purification system equipped with a UV lamp providing water resistivity >18 MOhm cm). Immediately afterwards, the gold crystal was annealed in a hydrogen flame till it became red hot for 2 min followed by immediate quenching in hydrogen-saturated ultraclean water while it was still hot and dark red in colour. Finally, the crystal was dried under a stream of high-purity argon. The electrode was then immersed in THF solution containing 0.05 mM of carbo -mer for molecular assembly. After 1 min, modified electrodes were thoroughly rinsed with solvent (THF) following removal from the assembly solution, before single molecule resistance measurements. A Teflon liquid cell and Teflon O-ring, pre-cleaned with the Piranha solution, were assembled on the Au(111) substrate electrode and 0.2 ml mesitylene or ionic liquid (Trihexyltetradecyl-phosphonium bis(2,4,4-trimethylphenyl)phosphinate) were added to the STM cell for STM break junction measurements. STM break junction experiments STM break junction experiments were carried out with a Molecular Imaging Picoscan or Picoplus scanning tunnelling microscope (Agilent). Current preamplifiers with gains of 1, 10 and 1,000 nA V −1 were used for measurements. The STM tips were mechanically cut gold wires (wire diameter=0.25 mm) and the substrate electrode was an Au(111) disk single crystal prepared as described above. The experimental procedure was to use the STM software to drive the tip to approach the molecule-modified electrode with preset parameters, typically a bias voltage of 0.1 V and a tunnelling setpoint of 0.1 nA. After the STM tip was engaged, the electrode surface was first imaged by STM in constant current mode, confirming a clean surface and a sharp tip. Before the measurement of single molecule conductance of the target molecules, the control experiment was typically performed using Au STM tips and Au substrate electrodes in pure solvent without adding molecules. What we observed is that there are current steps in individual current–distance traces ( Supplementary Fig. 2a ), with a value of ~3,850 and 7,700 nA for a bias voltage of 0.05 V. These currents divided by the bias voltage give the conductance values of 77,000 and 154,000 nS, corresponding to quantized conductance one and two G 0 , respectively, associated with Au atomic junctions [26] (peaks in Supplementary Fig. 2b ). Then, the STM feedback loop was switched off and the STM was programmed to move the tip in and out of contact with the surface. The tip movement speed was typically 10–20 nm s −1 . During the process of the formation and breaking of junctions, molecules may bridge across the two electrodes (the gold STM tip and gold substrate) via the amine-anchoring groups of molecules. The tip was then retracted to break the molecular junctions and the current versus distance traces were recorded during the tip-retracting process. The displacement of the tip was automatically repeated to generate a large number of current versus distance traces. 10,000–20,000 current–distance traces were recorded at a given bias for statistical analysis and typically three bias voltages ( V bias ) were measured ( Supplementary Figs 3 and 4 ). The junction current increases proportionally to V bias , showing a quasi-linear bias dependence. Unless specifically mentioned, all histograms were constructed using all the measured traces without selection. As an example, Supplementary Fig. 5 shows all-data histograms for carbo-n-butadiene (DBA) B from six different experiments measured at a bias voltage of 0.1 V. Each histogram was constructed from 1,000 current–distance traces without data selection. For electrochemical gating experiments, the data points with error bars shown in Fig. 5d are averaged from different experiments measured on different days. On average, each data point (potential) was obtained from at least three measurements, and some data points are averaged from up to 10 measurements. Often, we started measuring from zero gating potential, and then went to negative potential. Each potential was measured at least twice (collecting ~2,000 individual traces) and then we went to another potential. After measuring negative potentials, we also re-measured (to check) the potential around 0.0 V, which was measured a couple of hours previously. Measurements carried out on different days show consistent conductance values. Our extensive measurements in mesitylene and in ionic liquid show that there is no solvent effect in this study. [44] Electron transport calculations The structures of the molecular junctions were relaxed as follows. For carbo -benzene A , a periodic system was constructed as shown in Supplementary Fig. 6a , which contains the molecule bridging two Au electrodes. The bonding of the molecule to either electrode occurs via the lone pair of the N atom with an Au adatom at the tip of the electrode apex. During the structure relaxations, all atoms in the molecule and the Au apexes were allowed to relax, while the surface Au atoms were frozen to their bulk Au(111) crystal structure positions (the plane of Au atoms nearest to the left of the simulation box). Relaxations were carried out for various electrode–electrode separations to identify the lowest energy geometry, which was 35.7 Å between the Au surfaces. The relaxations for the graphene flake system were carried out in a similar manner. For the DBA B systems, the minimum energy electrode–electrode (Au surface to surface) separation was set to 35.3 Å, which is an intermediate between the ideal separation for the molecule having a dihedral of 0° and 180°. The various conformations were determined by fixing the coordinates of the Si atoms (displayed as blue atoms in Supplementary Fig. 6b ) while allowing all other atoms to relax. The structure relaxations were carried out using the Vienna ab initio simulation package (VASP) [45] , [46] with the projector augmented-wave potentials [47] and using the Perdew–Burke–Ernzerhof generalized gradient approximation (PBE-GGA) [48] . The kinetic energy cutoff of the plane wave basis was set to 400 eV. The relaxation was carried out until the force on all atoms that were free to relax was less than 0.01 eV Å −1 (VASP input files are provided in Supplementary Note 1 ). For each structure that was relaxed ( carbo -benzene, graphene flake, DBA having various dihedral angles) between Au electrodes, two-probe structures were constructed to calculate the electron transmission through each system. This was carried out by extending the electrodes by placing Au atoms at their appropriate crystal lattice positions, resulting in a two-probe structure, as shown in Fig. 7 . Atomic coordinates ( xyz format) of all two-probe structures are available in the Supplementary Information . Note that bulk electrodes were used. The two-probe structure can be partitioned into three regions: the central region containing the molecule and parts of each electrode, and the right and left electrodes that extend to infinity in either direction. The electron transmission through such systems can be calculated with the NEGF formalism within the DFT (NEGF-DFT) framework [30] , [31] . In this work, the Nanodcal implementation of NEGF-DFT was used (‘Nanoacademic Technologies’ http://nanoacademic.ca , accessed: 5 February 2014). Interested readers are directed to refs 30 , 31 , 32 , 33 where the technique has been extensively described. The retarded Green’s function at energy E is G ( E )=[ES− H −∑ 1 −∑ 2 ] −1 , where H and S are the Hamiltonian and overlap matrices of the central region, and ∑ 1,2 are the self-energies representing the influence of the two electrodes on the central region. The self-energies are complex quantities with the real part representing the shift and the imaginary part representing the broadening of the energy levels in the central region in response to the presence of the electrodes. The broadening effect of each electrode can be expressed as the broadening matrix, . The electronic density matrix for the central region is calculated as , with μ 1,2 being the electrochemical potentials of the two electrodes and f ( E , μ ) is the Fermi-Dirac function. The density, ρ , is used to seed a subsequent DFT step, yielding a new H to input into another Green’s function step, and the process is repeated until self-consistency is achieved. The transmission function can then be obtained from the Green’s function as T( E )=Tr(Γ 1 G Γ 2 G † ). This gives the probability of an electron with a given energy passing from electrode 1 through the molecule and into electrode 2. The low-bias conductance of the molecule can be approximated by the transmission at the Fermi level, E F , of the electrodes multiplied by the quantum of conductance, G 0 =(2 e 2 / h ). The gate calculations are performed by setting up a system as shown in Fig. 6a . The gate is applied on one side of the central region simulation box by setting up a gate-induced electrostatic boundary condition for the Hartree potential when solving the Poisson equation. In Fig. 6a , the box dimension in the vertical dimension is 26 Å, and the molecule is near the middle. Therefore, the atoms of the molecule are ~13 Å from the gate (some are closer, some are farther). For the numerical electron transport calculations, the valence electrons of Au were treated with single-ζ polarized basis sets and all other elements were treated with double-ζ polarized basis sets. The atomic cores were described with Troullier–Martins norm-conserving pseudopotentials [49] . The PBE-GGA was used for the exchange-correlation functional [48] . A real-space grid with more than five points per Å was used to describe the basis. For the reciprocal space, the Brillouin zone was sampled with 2 × 2 k -points in the transverse dimension (perpendicular to transport direction), which was sufficient since the cell had transverse vectors of 26.5 Å × 26.5 Å. We note here that some groups apply a shift to the energy of the occupied and unoccupied molecular orbitals to account for self-interaction errors in the DFT description [50] . This approach has been found to be essential in obtaining quantitative predictions of conductance [51] . While we agree that applying such techniques may help us make more quantitative predictions, we feel it is not necessary for our comparative qualitative computations. All our results involve a comparison of systems and we make no claims in terms of actual conductance values based on the calculations. The conclusions of our comparisons will not be affected by the exact positions of the frontier molecular orbitals. It is worth commenting on the suitability of structures relaxed with projector augmented-wave potentials for electron transport calculations employing Troullier–Martins norm-conserving pseudopotentials. Several studies have determined that structure relaxations yield very similar results with the two methods as long as the same functional is used [52] , [53] , [54] , [55] . In this work, the PBE-GGA functional was used for both the structure relaxations and the electron transport calculations (Nanodcal input files are provided in Supplementary Note 1 ). Dihedral angle potential energy profile The rotational profile about a DBA molecule in vacuum ( Fig. 8 ) has been calculated with B3LYP/6-31G(d). The energy of the molecule as the dihedral angle (marked in Fig. 8a ) is changed and plotted in Fig. 8b . The global energy minimum is near 180°. Note that the other planar conformation (0°) is not a local minimum because of the steric effects of the large TIPS groups. Instead, there is a local minimum near 45°. The rotational energy barrier between these minima is over 75 meV, which is nearly three times the thermal energy available at room temperature. Therefore, we expect a DBA molecule (in vacuum, not connected to electrodes) to be found in one of these conformational minima. However, this potential energy surface may change once the molecule is anchored to electrodes and interacting with solvent. In any case, the purpose of Fig. 4 is to illustrate how rotation about a single bond can affect transmission. There are certainly other factors affecting the transmission. For example, the specific geometry at the amine–gold interface can have an important influence on the conductance/transmission [56] . How to cite this article: Li, Z. et al. Towards graphyne molecular electronics. Nat. Commun. 6:6321 doi: 10.1038/ncomms7321 (2015).